In-situatomic-scale observation of irradiation-induced void formation The formation of voids in an irradiated material significantly degrades its physical and mechanical properties. Void nucleation and growth involve discrete atomic-scale processes that, unfortunately, are not yet well understood due to the lack of direct experimental examination. Here we report an in-situ atomic-scale observation of the nucleation and growth of voids in hexagonal close-packed magnesium under electron irradiation. The voids are found to first grow into a plate-like shape, followed by a gradual transition to a nearly equiaxial geometry. Using atomistic simulations, we show that the initial growth in length is controlled by slow nucleation kinetics of vacancy layers on basal facets and anisotropic vacancy diffusivity. The subsequent thickness growth is driven by thermodynamics to reduce surface energy. These experiments represent unprecedented resolution and characterization of void nucleation and growth under irradiation, and might help with understanding the irradiation damage of other hexagonal close-packed materials. Irradiation resistance is one of the critical material properties that is important for many applications including nuclear energy [1] , [2] , [3] , [4] , outer space systems [5] and other industrial applications [6] , [7] . Materials under irradiation of high-energy particles, such as neutrons, ions and electrons, will develop point defects or defect clusters, which may subsequently evolve into microstructural flaws, such as voids, dislocation loops, solute segregation or precipitation [3] , [8] , [9] , [10] , [11] , [12] . Such defects and flaws not only deteriorate the physical properties of irradiated materials, but also cause direct structural failure. In particular, the void formation will lead to volumetric swelling and eventual failure. Voids could form in almost all materials under irradiation [8] , [9] , [13] , [14] , [15] , [16] , [17] , [18] , [19] , [20] . They nucleate from the agglomeration of mobile vacancies, and evolve with the absorption and emission of vacancies or self-interstitials at the void surfaces [21] . In many cases, they appear as a polyhedron bounded by several low-energy flat surfaces. Experimental investigations reported so far have concentrated on void growth behaviours, such as void growth rate, size and spatial distribution [9] , [13] , [15] , [21] , [22] , [23] , [24] . Although attempts have been made to observe void formation [23] , [25] , [26] , no atomic-scale observation of void nucleation and early growth has been reported because of experimental difficulties. The lack of understanding of void formation behaviour at the atomic scale has adversely affected the development of advanced theoretical models to predict void evolution under irradiation. This is evidenced by the fact that existing models [27] , [28] , [29] , [30] , [31] , [32] , [33] , [34] , [35] , [36] , [37] cannot accurately predict the void evolution at the atomic level that is experimentally observed in the current study. Specifically, it is observed here that the void formation is largely controlled by the atomic process on the void surfaces, a phenomenon that has not been reported before and can only be observed in situ at atomic scale. A fundamental understanding of the void formation mechanism is of both scientific and technical importance to advance the design of new irradiation-resistant materials. Here we report an in-situ observation of the nucleation and early growth mechanisms of voids in Mg at the atomic scale. Mg is chosen as a model hexagonal close-packed (hcp) material. This is motivated primarily by its low-melting point and very-low-electron damage threshold of 100 kV (refs 38 , 39 , 40 ), making it feasible to use high-resolution transmission electron microscopy (HRTEM) to simultaneously induce electron irradiation damage and to observe the resulting damage evolution in situ at atomic scale in a commercial electron microscope operating at 200 kV at room temperature. Void nucleation and early length growth We observed that under electron irradiation, self-interstitial atom (SIA) loops first form on basal planes in the grain interior. Subsequently, voids nucleate in the vicinity of these SIA loops, which act as biased sinks for SIAs, thus creating an adjacent vacancy supersaturation zone [21] , as shown in Fig. 1a . In addition, SIAs may also diffuse to free surface of the transmission electron microscopy (TEM) foil (70 nm in thickness), which helps enhance the excess vacancy concentration. The void nuclei observed here usually have a thickness of 1.0–1.6 nm (four to six atomic layers and 0.26 nm per layer) and a length of 3.0–4.0 nm. Some small voids are observed to appear for a short period of time and then disappear (see Supplementary Movie 1 ), which suggests the existence of a critical nucleus size, below which the void is not stable. This also indicates that the void nucleation is a thermally activated process that is similar to the nucleation process in a phase transformation. After their nucleation, voids first grew in two dimensions on the basal plane ( a direction, hereafter referred to as Stage 1) and then thicken in the direction perpendicular to the basal plane ( c direction, hereafter referred to as Stage 2). The Stage 1 is demonstrated by a series of still images, Fig. 1b–d , picked sequentially from an in-situ HRTEM video (see Supplementary Movie 2 ). As shown, the void grew to the SIA loop edge but did not grow beyond it. The thickness of the void did not change in this stage (about 1.56 nm or six atomic layers), whereas the length grew to 15–20 nm. The elongated void morphology in Fig. 1d is similar to that observed in electron-irradiated zirconium [23] , [41] , which was pre-irradiated by fast neutrons. It should be noted that the voids have a plate-like polyhedron shape in three dimensions with their broad face on the (0001) basal plane. Our HRTEM images and videos were taken along an orientation, which resulted in two-dimensional images with void thickness along the c -axis and length on the basal plane (see Fig. 4 and Supplementary Fig. S1 ). For simplicity, the void dimension on the basal plane is hereafter referred to as void length. 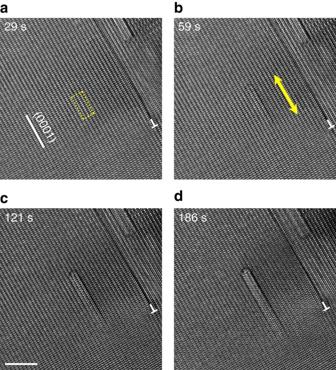Figure 1: A series of HRTEM images of void length growth under electron irradiation. (a) A void (outlined by dashed lines) nucleated near the interstitial dislocation loop. (b–d) Stage 1 growth of the void, where it grew in length but not in thickness. The length growth direction is indicated by the yellow arrow. Detailed growth process is shown inSupplementary Movie 2. The specimen is irradiated over a dose range of 0.95–1.17 displacement-per-atom (d.p.a.). Scale bar, 5 nm. Figure 1: A series of HRTEM images of void length growth under electron irradiation. ( a ) A void (outlined by dashed lines) nucleated near the interstitial dislocation loop. ( b – d ) Stage 1 growth of the void, where it grew in length but not in thickness. The length growth direction is indicated by the yellow arrow. Detailed growth process is shown in Supplementary Movie 2 . The specimen is irradiated over a dose range of 0.95–1.17 displacement-per-atom (d.p.a.). Scale bar, 5 nm. Full size image Void thickness growth In the Stage 2, voids started to grow in thickness. This growth process is found to be discrete, rather than smooth and continuous, whereby the void thickness grew one vacancy layer at a time. This is demonstrated in a typical void growth evolution shown in Fig. 2 . First, a vacancy layer nucleated on a basal plane that is adjacent to the void surface and near the centre of the void’s (0001) facet, as marked by the yellow arrow in Fig. 2a . After its nucleation, it takes this vacancy layer about 20 s to spread over the whole (0001) facet, making the void one atomic plane (~0.26 nm) thicker ( Fig. 2b,c ). However, it takes another 50 s to nucleate the next vacancy layer near the centre of the (0001) facet ( Fig. 2d ). This process as described above can be viewed in Supplementary Movie 3 . 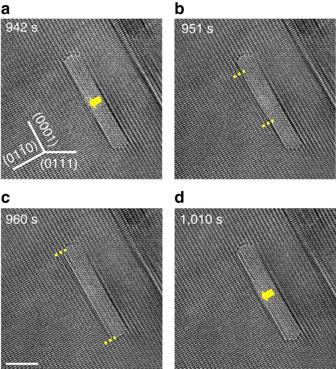Figure 2: Void thickness growth in Stage 2 over a dose range of 2.27 to 2.36 d.p.a. (a) First vacancy layer nucleates on the top of the (0001) facet as indicated by the yellow arrow. (b) The spreading of the vacancy layer on the (0001) facet, the size of the vacancy layer is designated by the dashed lines. (c) Vacancy layer extends over the whole (0001) facet surface. (d) Subsequent nucleation of a new vacancy layer (seeSupplementary Movie 3for more details). Scale bar, 5 nm. Figure 2: Void thickness growth in Stage 2 over a dose range of 2.27 to 2.36 d.p.a. ( a ) First vacancy layer nucleates on the top of the (0001) facet as indicated by the yellow arrow. ( b ) The spreading of the vacancy layer on the (0001) facet, the size of the vacancy layer is designated by the dashed lines. ( c ) Vacancy layer extends over the whole (0001) facet surface. ( d ) Subsequent nucleation of a new vacancy layer (see Supplementary Movie 3 for more details). Scale bar, 5 nm. Full size image As the void thickens, its side facets grow larger, as shown in Fig. 3 . The sidewalls of the void are composed of facets when the thickness is small ( Fig. 4a ); and facets appear when the thickness is larger ( Fig. 4b ). The void length growth occurs slowly via vacancy layer nucleation and growth on the sidewalls in this stage. The growth of the sidewalls starts with the nucleation of a vacancy layer on a facet at its intersection with the (0001) basal facet as marked in Fig. 3b . The vacancy layer extends its size on the facet ( Fig. 3c ) until it reaches the other corner bounded by the facet ( Fig. 3d ), which enlarges the facet area by one atomic layer. This process grows the facet without growing the void in the length direction. Further void growth in this direction needs the formation of a vacancy layer on the facet directly (see Supplementary Movie 3 ). 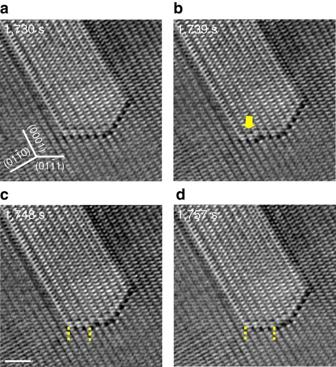Figure 3: Formation of void side facets over a dose range of 3.37 to 3.41 d.p.a. (a) Facet plane indexes. (b) A vacancy layer nucleated on thefacet near its intersection with the (0001) facet as indicated by the yellow arrow. (c) The vacancy layer extended on thefacet, which leads tod, the growth of thefacet in the thickness direction. SeeSupplementary Movie 3for more details. Scale bar, 2 nm. Figure 3: Formation of void side facets over a dose range of 3.37 to 3.41 d.p.a. ( a ) Facet plane indexes. ( b ) A vacancy layer nucleated on the facet near its intersection with the (0001) facet as indicated by the yellow arrow. ( c ) The vacancy layer extended on the facet, which leads to d , the growth of the facet in the thickness direction. See Supplementary Movie 3 for more details. Scale bar, 2 nm. 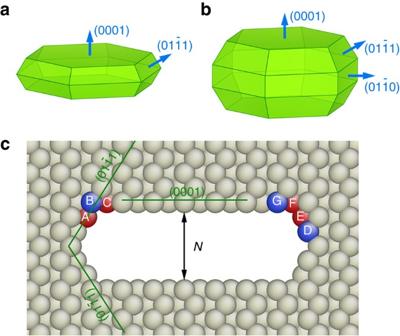Figure 4: Void shape and vacancy inter-facet diffusion paths. (a) Illustration of three-dimensional geometry and facet indexes of a void with small thickness bounded by {0001} andfacets. (b) Geometry and facet indexes of a void with larger thickness bounded by {0001},andfacets. (c) Atomic configuration for vacancy diffusion paths between a (0001) facet and thefacets (A-B-C or D-E-F-G) for a five-atomic-layer-thick void (N=5). The image is projected along adirection. Two possible different diffusion paths are considered due to the double lattice structure in hcp49. Full size image Figure 4: Void shape and vacancy inter-facet diffusion paths. ( a ) Illustration of three-dimensional geometry and facet indexes of a void with small thickness bounded by {0001} and facets. ( b ) Geometry and facet indexes of a void with larger thickness bounded by {0001}, and facets. ( c ) Atomic configuration for vacancy diffusion paths between a (0001) facet and the facets (A-B-C or D-E-F-G) for a five-atomic-layer-thick void ( N =5). The image is projected along a direction. Two possible different diffusion paths are considered due to the double lattice structure in hcp [49] . Full size image The voids have a polyhedral geometry bounded by {0001}, and facets after the Stage 2 growth, as determined by viewing the voids along , <0001> and zone axes (see Supplementary Fig. S1 ). This is consistent with the void morphology in magnesium observed under neutron irradiation [14] . Given the fact that the surface energies of the {0001} and surfaces are similar, and slightly lower than that of [42] , [43] , the equilibrium void shape should be approximately equiaxed [14] , [43] . However, the early-stage voids observed here are mostly plate-shaped with their thickness much smaller than their length. The formation energy calculation shows that the plate-shaped voids are less stable than that in near equiaxed voids in a similar volume size (see Supplementary Fig. S2 ). Therefore, the geometry of the voids observed here is not in thermodynamic equilibrium. The observed non-equilibrium void geometry is caused by their anisotropic growth kinetics. The void length is measured to grow at a speed of ~2.8 nm min −1 at the Stage 1, which is more than an order of magnitude faster than the growth in the thickness direction, ~0.2 nm min −1 , as observed in the Stage 2 (see Supplementary Fig. S3 for more details). The thickening of the void in the Stage 2 is driven by thermodynamics, that is, the reduction of the total surface energy, which favours a near-equiaxed void geometry. The slow growth kinetics in the thickness direction is caused by both the void growth mechanism and the anisotropic diffusion kinetics of vacancies. Figure 2 shows that it takes 50 s to nucleate a new vacancy layer on the (0001) void facet, which is about 2.5 times longer than the time it takes for the vacancy layer to extend across the whole facet. This suggests that the slow growth kinetics in the thickness direction is primarily caused by the difficulty in vacancy layer nucleation, which is similar to what was predicted in silicon [44] . Furthermore, vacancies diffuse along a directions about two times faster than along c directions at room temperature [45] , [46] . Therefore, a higher flux of vacancies will flow to and sidewalls than to the {0001} facets. This diffusion anisotropy is therefore partially responsible for the slow growth in the c direction. Energy barriers for vacancy inter-facet diffusion To help understand the void growth behaviour further, the energy barriers for the vacancy diffusion between a basal (0001) facet and side facets are calculated by means of molecular dynamics (MD) simulation using the nudged-elastic-band method [47] and an empirical potential developed by Liu et al. [48] Because of the double lattice structure of hcp crystals [49] , there are two possible diffusion paths for vacancy to diffuse between the {0001} and facets, that is, A-B-C and D-E-F-G paths as shown in Fig 4c . 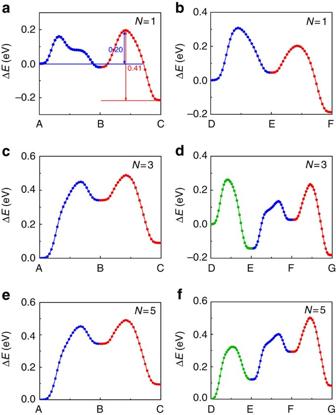Figure 5: Free energy change of a vacancy along inter-facet diffusion paths. (a,b) Diffusion paths A-B-C and D-E-F with void thicknessN=1, respectively. (c,d) Diffusion path A-B-C and D-E-F-G withN=3, respectively. (e,f)N=5. The vacancy inter-facet diffusion barrier along the whole diffusion path is estimated as the difference between maximum potential energy and that of the initial configuration. For example, the overall barrier for A→B→C path is determined as 0.20 eV (blue arrow), and the barrier for the reverse path C→B→A is 0.41 eV (red arrow). Note that when a void is one-atomic-layer thick (N=1), position G does not exist in the atomic configuration. Figure 5 shows the calculated free energy change along the diffusion paths A-B-C and D-E-F-G for different void thickness. As shown, there are several energy barriers along each diffusion path, with the highest one limiting the overall diffusion rate along the path. For instance, as indicated by the arrow in Fig. 5 , the barrier for the A→B→C path is determined as 0.20 eV, whereas a larger barrier for the reverse path C→B→A is 0.41 eV, suggesting that the net vacancy diffusion direction should be A→B→C. As shown in Fig. 4c , symbols A→B→C and D→E→F→G represent vacancy diffusion paths from facets to {0001} facets, hereafter referred to as the forward diffusion, whereas C→B→A and G→F→E→D represent reverse diffusion paths. The corresponding energy barriers for the forward and reverse diffusions are illustrated in Fig. 6 . Figure 5: Free energy change of a vacancy along inter-facet diffusion paths. ( a , b ) Diffusion paths A-B-C and D-E-F with void thickness N =1, respectively. ( c , d ) Diffusion path A-B-C and D-E-F-G with N =3, respectively. ( e , f ) N =5. The vacancy inter-facet diffusion barrier along the whole diffusion path is estimated as the difference between maximum potential energy and that of the initial configuration. For example, the overall barrier for A→B→C path is determined as 0.20 eV (blue arrow), and the barrier for the reverse path C→B→A is 0.41 eV (red arrow). Note that when a void is one-atomic-layer thick ( N =1), position G does not exist in the atomic configuration. 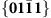Figure 6: Energy barriers for vacancy diffusion between {0001} andfacets. (a) Energy barriers for forward diffusion along the path A→B→C and its reverse diffusion (C→B→A) as a function of void thicknessN. (b) Energy barriers for forward diffusion along the path D→E→F→G and its reverse diffusion (G→F→E→D). Full size image Figure 6: Energy barriers for vacancy diffusion between {0001} and facets. ( a ) Energy barriers for forward diffusion along the path A→B→C and its reverse diffusion (C→B→A) as a function of void thickness N . ( b ) Energy barriers for forward diffusion along the path D→E→F→G and its reverse diffusion (G→F→E→D). Full size image Figure 6 shows that when the void is over five atomic layers thick, the energy barriers for the reverse vacancy diffusion (C→B→A and G→F→E→D) are smaller than those for the forward diffusion (see Fig. 6 ). As a result, vacancies will diffuse from {0001} facets to facets to help voids to grow in length, which is consistent with the experimental observation in the Stage 1. It should be noted that, during the Stage 2 growth, the diffusion energy barrier effect is overwhelmed by the thermodynamic effect, where the voids grow in thickness to reduce the total surface area and to lower the overall Gibbs free energy. The diffusion of vacancies along the path of C→B→A and G→F→E→D also helps to explain the nucleation location of the vacancy layer on the {0001} and facets. As vacancies diffuse from the edge of a (0001) facet to the edges of intersecting facets, vacancies will be depleted in the region near the edge of the (0001) facet, making it nearly impossible for vacancy layer to nucleate in these regions, because a supersaturation of vacancies is the prerequisite for the nucleation of a new vacancy layer. This is why the vacancy layer always nucleates near the centre of the {0001} facets, as observed in Fig. 2 . On the other hand, the vacancy diffusion leads to the supersaturation of vacancies near the edges of the facets, which promotes the vacancy layer formation, as observed experimentally in Fig. 3 . The vacancy diffusion from {0001} facets to facets also contributed to the observed maintenance of void thickness during the Stage 1 growth. In this stage, as the area of a {0001} facet is relatively small, the vacancy diffusion from the {0001} facets to the facets depletes vacancies on the {0001} facets, making it difficult to nucleate a new vacancy layer on the {0001} facets. This will suppress the thickening of the void until it grows laterally to a size larger than a critical value. At this critical size, vacancies near the centre area of the {0001} facets are able to accumulate to a supersaturated state to nucleate a vacancy layer, which transits the Stage 1 length growth to the Stage 2 thickness growth. Figure 6 also shows that before the void nucleus reaches a critical thickness, the diffusion barriers for the forward diffusion A→B→C and D→E→F→G are lower than their reverse diffusions. In other words, more vacancies will diffuse from the sidewalls to the {0001} facets. This could help the void to thicken to a critical value at the Stage 1. The transition of the diffusion barriers could be closely related to the geometrical change for the atomic configurations of the void in terms of the number of atomic layers or void thickness. The thickness-dependent inter-facet diffusion barriers for vacancies here are quite similar to the three-dimensional Ehrlich–Schwoebel barriers for the surface adatoms diffusion [50] . As seen in Supplementary Fig. S2 , a void nucleus with a thickness of a few atomic layers is energetically more stable than a basal plane vacancy dislocation loop when the total number of vacancies is small. Similar calculation results are also reported for α-Zirconium [51] , [52] . This suggests that a void with a thickness of a few atomic layers should not collapse when the total number of vacancies is small. Our in-situ HRTEM observation revealed for the first time the irradiation-induced void nucleation and growth at the atomic scale. Under irradiation, interstitial loops form first, producing supersaturated vacancy zones in their vicinity, where voids are nucleated. A void nucleus larger than a critical size will grow in the length direction first (Stage 1) and then in thickness (Stage 2). These observations may help us with the understanding of void formation of other hcp systems or under other irradiation conditions. For example, the void thickness growth in the Stage 2 observed here is similar to what was observed in Zr via low-resolution TEM under high-voltage electron irradiation (1 MeV) at elevated temperature (573 K) [23] , [41] . Although the void nucleation and early growth process in Zr has not been reported, it might be similar to what we have observed in Mg. This needs further studies to clarify. The shape of the void in Mg is observed as a polyhedron bounded with {0001}, and facets under electron irradiation. The same void geometry was observed for facet voids in Mg under neutron irradiation [14] . Interestingly, similar morphology of faceted voids were also found in other hcp materials, such as Ti [20] and Zr [41] , although fast neutrons produce defects in a manner that is very different from those by electrons. Therefore, the void formation mechanisms observed here could potentially help with the understanding of void formation in other hcp materials and/or under other irradiation conditions, and may inspire new ideas with the development of better predictive modelling. TEM sample preparation Magnesium with 99.9% purity was used in this investigation. The major impurity elements are Fe=0.0510 wt%, Mn=0.0320 wt%, C=0.0089 wt%, Al=0.0054 wt%, Na=0.0027 wt%, Zn=0.0026 wt%, H=0.0010 wt% and O=0.0007 wt%. TEM foil was electro-polished in a solution of 5.3 g lithium chloride, 11.16 g magnesium perchlorate, 100 ml 2-butoxy-ethanol and 500 ml methanol at −30 °C and 200 mA, then low energy ion-milled on a cold stage and plasma cleaned for HRTEM observation. Thickness measurement The sample thickness in the irradiated region is close to 70 nm as determined by electron energy-loss spectra (EELS) using the log-ratio method [53] , given as t / λ =ln( I t / I 0 ), where λ is the inelastic scattering mean free path ( λ =150 nm for Mg [54] ), I 0 and I t are the total area under the zero-loss peak and the whole spectra, respectively (see Supplementary Fig. S4 ). Electron irradiation conditions The electron irradiation and in-situ observation were performed in a JEM-2010F transmission electron microscope operating at 200 kV at room temperature. The electron beam current is about 8.2 × 10 23 e m −2 s −1 , which corresponds to a damage rate of ~1.4 × 10 −3 displacement-per-atom (d.p.a.) s −1 . The void in Fig. 1 nucleated at a dose of around 0.95 d.p.a. The listed times in Figs 1 , 2 , 3 are times from the starts of video recording and are listed in Supplementary Movies 2 and 3 . Similar void growth behaviour is observed in samples with various thickness (105, 155, 195, 300 and 460 nm), as shown in Supplementary Figs S5–S7 . Energy barrier calculation To calculate the energy barriers for vacancy inter-facet diffusion, a periodic simulation cell with the size of 6.0 × 6.0 × 1.6 nm 3 along the x ( ), y ([0001]) and z ( ) directions is used. The system size has been tested with negligible size effect on the results. A centre void is created along the z direction with the side surfaces being (0001), and . The length of the void along x is about 3.0 nm and the thickness N along z increases from one to nine atomic layers to study the effect of thickness. The interatomic interaction is described by the embedded atom method potential developed by Liu et al. [48] , which well reproduces the surface formation energy and vacancy formation energy with reference to experiments. After relaxing the simulation cell, the barrier is calculated at 0 K using the nudged-elastic-band method [47] . Formation energy calculation The formation energies are calculated using MD simulations with the same embedded atom method potential developed by Liu et al. [48] For all configurations, the simulation cells are first equilibrated at 300 K until the potential energy converges. The temperature is then quenched down to 0 K for the energy calculation. The specific formation energy is defined as =(E total − N A E coh )/ N v . In the equation, E total is the total potential energy of the system with N A atoms and N v vacancies. E coh is the cohesive energy of hcp Mg. How to cite this article: Xu, W. et al. In-situ atomic-scale observation of irradiation-induced void formation. Nat. Commun. 4:2288 doi: 10.1038/ncomms3288 (2013).